Revealing the role of defects in ferroelectric switching with atomic resolution Ferroelectric materials are characterized by a spontaneous polarization, which can be reoriented with an applied electric field. The switching between polarized domains is mediated by nanoscale defects. Understanding the role of defects in ferroelectric switching is critical for practical applications such as non-volatile memories. This is especially the case for ferroelectric nanostructures and thin films in which the entire switching volume is proximate to a defective surface. Here we report the nanoscale ferroelectric switching of a tetragonal PbZr 0.2 Ti 0.8 O 3 thin film under an applied electric field using in situ transmission electron microscopy. We found that the intrinsic electric fields formed at ferroelectric/electrode interfaces determine the nucleation sites and growth rates of ferroelectric domains and the orientation and mobility of domain walls, whereas dislocations exert a weak pinning force on domain wall motion. The ability of an electric field to switch the spontaneous polarization in a crystal between energetically degenerate orientation states is the defining characteristic of a ferroelectric material and provides the underlying storage mechanism in an important class of non-volatile memories [1] , [2] . This switchable polarization couples with electronic transport properties [3] , [4] , [5] , [6] , surface chemistry [7] , strain and magnetic order [8] , [9] , enabling multifunctional devices. The switching of the spontaneous polarization occurs via the nucleation and growth of favourably oriented domains through a highly inhomogeneous process, whereby local variations in free energy, caused by defects, dominate switching kinetics [10] . Macroscale ferroelectric switching models aggregate this behaviour [11] , but a specific understanding of the role of defects is necessary to engineer ferroelectric devices, including mollifying fatigue, imprint and ageing effects [11] , [12] , and to scale devices down to the size of the defect spacing where a statistical treatment is not applicable. Defects within ferroelectric materials are generally classified into two non-mutually exclusive categories based on their influence on the free-energy diagram. Random-field defects break the degeneracy of the polarization states to favour one or more orientations. Random-bond defects change the barrier height for transitions between degenerate states. The most prominent and voluminous defects in planar thin film heterostructures are the two interfaces, which not only break the crystal symmetry, but also are accompanied by physical and chemical reconstructions, bound charges, space charges and strain. These interfaces and defects existing in the ferroelectric film determine the characteristics of ferroelectric switching, as has been demonstrated by switching spectroscopy piezoresponse force microscopy [10] , [13] . The effects of the random-field and random-bond defects are manifested by changes in nucleation biases of the local switching under the surface probe. A direct correlation to the physical defects underlying such behaviour is, however, absent. In contrast, the atomic resolution afforded by contemporary aberration-corrected transmission electron microscopy (TEM) is ideal for characterizing crystalline defects and following the ferroelectric switching process in situ . There are, however, only a handful of TEM studies of ferroelectric domain switching in bulk crystals [14] , [15] , [16] . The direct characterization of ferroelectric switching in thin-film heterostructures is now possible with the recent integration of scanning probe and TEM [17] , [18] . Here we report real-time TEM observations of nanoscale ferroelectric switching along the cross-section of a PbZr 0.2 Ti 0.8 O 3 (PZT) film to reveal the role of defects, specifically the interfaces and threading dislocations, in polarization switching behaviour. The domain wall motion along the film normal, inaccessible by surface probing techniques, can be directly followed by using in situ TEM, providing insight into the switching in nanoscale ferroelectric heterostructures, which comprise most ferroelectric devices. Despite the localized electric field concentration at the tip contact, the domain nucleation site(s) and voltage is dictated by the built-in electric fields formed by Schottky junctions between the ferroelectric film and electrodes. These intrinsic fields also result in a significant asymmetry in domain wall mobility. It was found that dislocations show a weak pinning effect on the domain wall motion; nevertheless, the switching processes are primarily controlled by the interfaces. 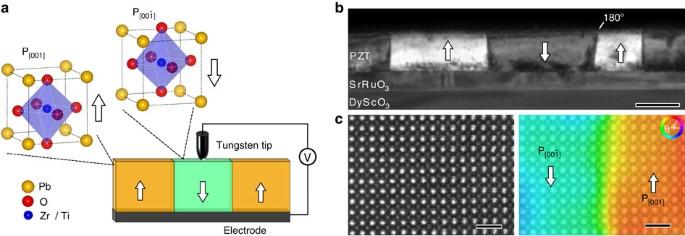Figure 1: Polarization switching viain situTEM. (a) Schematic of the formation of a downward polarized (P[00[macr1]]) region within an upward polarized (P[001]) film cross-section by the application of a local electric field via a surface probe. The polarization results from the offset of the oxygen octahedra to the Zr/Ti and Pb cations forming an electric dipole, which reorients upon switching. (b) A dark-field TEM image of alternatingP[00[macr1]]andP[001]domains produced in a 100-nm PZT film byin situelectrical switching. Scale bar, 100 nm. (c) A high-resolution high-angle annular dark-field image of the domain wall bordering a switched domain and the corresponding map of the polarization direction determined by the relative offset of the Zr/Ti atoms, confirming a 180° rotation. Scale bar, 1 nm. In situ ferroelectric switching In situ ferroelectric switching of a 100 nm PZT thin film was performed by applying a bias between a tungsten surface probe and a SrRuO 3 (SRO) bottom electrode as shown schematically in Figure 1a . PZT is a prominent displacive-type ferroelectric with a tetragonal perovskite structure. It has a spontaneous polarization along the [001] direction as a result of the relative displacement of the oxygen octahedra and Zr/Ti cations from their centrosymmetric positions. The PZT film was grown by 90° off-axis magnetron radio frequency sputtering [19] on a well lattice-matched (110) O DyScO 3 substrate (the subscript O denotes orthorhombic indices) with an epitaxial (110) O SRO bottom electrode [20] , [21] , resulting in a dislocation-free epitaxial c-axis-oriented PZT film ( Supplementary Fig. S1 ). When an applied electric field exceeds the coercive field, switching occurs by a 180° rotation of the polarization vector between upward P [001] and downward P [00[macr1]] states. The as-grown PZT film is initially polarized downward ( P [00[macr1]] ); the polarization vector pointing towards the bottom electrode, as determined by mapping the relative displacement vector between the Zr/Ti and Pb positions using aberration-corrected scanning TEM (STEM) [22] . A dark-field TEM image of switched P [001] (light) and P [00[macr1]] (dark) domains is shown in Figure 1b , whereas an atomic resolution high-angle annular dark field (HAADF) image at the domain wall and the corresponding polarization direction distribution is shown in Figure 1c confirming the 180° rotation of the polarization across the switched domain wall. Figure 1: Polarization switching via in situ TEM. ( a ) Schematic of the formation of a downward polarized ( P [00[macr1]] ) region within an upward polarized ( P [001] ) film cross-section by the application of a local electric field via a surface probe. The polarization results from the offset of the oxygen octahedra to the Zr/Ti and Pb cations forming an electric dipole, which reorients upon switching. ( b ) A dark-field TEM image of alternating P [00[macr1]] and P [001] domains produced in a 100-nm PZT film by in situ electrical switching. Scale bar, 100 nm. ( c ) A high-resolution high-angle annular dark-field image of the domain wall bordering a switched domain and the corresponding map of the polarization direction determined by the relative offset of the Zr/Ti atoms, confirming a 180° rotation. Scale bar, 1 nm. Full size image The domain formation process along both switching directions was analysed by real-time TEM imaging of the domain structure under a cyclic 0.1 Hz 18 V peak−peak triangle wave bias ( Supplementary Movie 1 ). This region of the PZT film was prepoled into the P [001] state after which a voltage ramp from 0 to 9 V was applied. 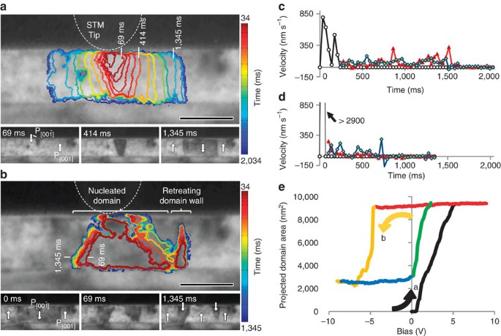Figure 2: Cyclic ferroelectric switching. This region of the PZT film, prepoled toP[001], undergoes cyclic switching using an 18 Vpeak−peaktriangle wave. (a) The negative and (b) positive switching branches are shown by contour plots of the domain outline versus time with selected corresponding TEM images shown below. (a) During the negative branch aP[00[macr1]]domain nucleates at the top surface and expands to a final width of ~250 nm. (b) On the subsequent positive branchP[001]domains nucleate at the bottom interface and expand across the film in a single time step. Scale bars, 100 nm. (c) Domain wall velocities for the negative switching branch along the vertical (black) and lateral (left-red and right-blue) directions. (d) Vertical and lateral domain wall velocities for the positive switching branch. (e) A ferroelectric hysteresis loop of domain area versus bias for the switching cycle containingaandb. The line colours in sequence correspond to the initial negative switching (black), negative saturation (red), positive switching (yellow), positive saturation (blue) and the second negative switching event (green). The 'negative' switching branch, that is, formation of a P [00[macr1]] domain by application of a negative electric field with a positive tip bias is shown in Figure 2a ( Supplementary Movie 2 ). The outward progression of the domain area from a nucleation site at the top surface is shown by a time-series of domain outlines accompanied by corresponding TEM images for the labelled 69, 414 and 1,345 ms cases. Onset of the P [00[macr1]] domain nucleation occurs at 0.4 V bias and initially proceeds by rapid growth along the applied field direction. Before reaching the opposite interface, the domain maintains a characteristic 'needle' geometry tapering to a point to reduce the area of the charged head-to-head domain wall at the leading edge. After reaching the opposite interface, the tapering of the domain walls, which produces small positive surface charge, relaxes to the vertical equilibrium (100) planes as they slowly propagate outward to a final domain width of ~250 nm. Figure 2: Cyclic ferroelectric switching. This region of the PZT film, prepoled to P [001] , undergoes cyclic switching using an 18 V peak−peak triangle wave. ( a ) The negative and ( b ) positive switching branches are shown by contour plots of the domain outline versus time with selected corresponding TEM images shown below. ( a ) During the negative branch a P [00[macr1]] domain nucleates at the top surface and expands to a final width of ~250 nm. ( b ) On the subsequent positive branch P [001] domains nucleate at the bottom interface and expand across the film in a single time step. Scale bars, 100 nm. ( c ) Domain wall velocities for the negative switching branch along the vertical (black) and lateral (left-red and right-blue) directions. ( d ) Vertical and lateral domain wall velocities for the positive switching branch. ( e ) A ferroelectric hysteresis loop of domain area versus bias for the switching cycle containing a and b . The line colours in sequence correspond to the initial negative switching (black), negative saturation (red), positive switching (yellow), positive saturation (blue) and the second negative switching event (green). Full size image For the subsequent 'positive' switching branch shown in Figure 2b , where the voltage is ramped from 0 to −9 V, a P [001] domain is formed within the previous P [00[macr1]] domain, but with very different kinetics than during negative switching. The nucleation of multiple P [001] domains occurs simultaneously at the bottom interface directly below the tip at −4.8 V after which the domains coalesce and expand to almost their full extent within a single 34 ms time step. Although this switching instance did not capture the P [001] nuclei at the bottom interface, several can be observed in the positive switching branch in Supplementary Movie 3 . In addition to this nucleated domain, there is a retreat of the rightmost edge of the surrounding P [00[macr1]] domain creating an additional region of P [001] formation labelled on the right side in Figure 2b . Limited lateral domain growth is observed, primarily on the right side, but it does not fully consume the surrounding P [00[macr1]] domain resulting in incomplete backswitching. The vertical and lateral domain wall velocities, determined by the forward edge and the mid-film domain wall position, respectively, are shown for the two switching paths in Figures 2c and d . Vertical switching during the positive branch is, however, a minimum of 3.6 times faster than the negative branch; this trend is reversed for the lateral creep rates, which favours the negative switching branch. These two processes were repeatable during subsequent switching cycles. Ferroelectric hysteresis The ferroelectric hysteresis loop for cyclic switching of the PZT film is shown in Figure 2e . The total switched domain area is used for the vertical axis rather than the classical 'polarization' derived from electrical measurements. This method is advantageous as it directly measures the property of interest, the region undergoing a change in spontaneous polarization, while ignoring leakage currents, dielectric contributions or electronic noise, which precludes electronic measurements in similarly small volumes. There are three obvious asymmetries in the hysteresis loop as follows: first, there is a horizontal shift of −2.2 V, corresponding primarily to a built-in electric field, and second, there is a vertical shift due to incomplete back switching. Third, as expected from the observed switching speeds, there is a large disparity in the slopes of the positive and negative switching branches. The translational offsets of the hysteresis loop are primarily the result of random-field defects, which can depend on the sample history [23] . Specifically, a portion of the observed loop translation is attributable to charged surface adsorbates and polar defects [24] , which have aligned to the as-grown P [00[macr1]] state, known as ageing. This effect favours the original P [00[macr1]] orientation, leading to a negative horizontal shift, and is a likely source of the incomplete backswitching. The asymmetry in the nucleation site and nucleation bias can be attributed to the built-in electric fields formed by Schottky junctions at the ferroelectric/electrode (semiconductor/metal) interfaces [25] , [26] , owing to the larger work functions of SRO and tungsten electrodes to the electron affinity of PZT [27] , [28] . The depletion of holes in p-type PZT near the electrodes ( Fig. 3a ) produces built-in electric fields ( E bi ), which reach their maximum at the interfaces (black line in Fig. 3b ). Given energy barriers for the W/PZT and SRO/PZT junctions of 1.3 and 0.9 V, respectively [27] , [28] , [29] , and assuming homogenous doping and full-carrier depletion corresponding to a doping concentration in a 100 nm film in excess of ~5×10 19 cm −3 , the built-in fields are −47.6 MV m −1 at the W/PZT interface and 39.6 MV m −1 at the SRO/PZT interface ( Supplementary Fig. S2 ). Under an external field ( E ext ), which for simplicity we momentarily assume to be homogenous, the total electrical field E total = E bi + E ext results in the largest positive field (favouring P [001] ) to occur at the PZT/SRO interface during positive switching and the largest negative field (favouring P [00[macr1]] ) at the PZT/W tip during negative switching, which corresponds exactly with the observed nucleation sites. 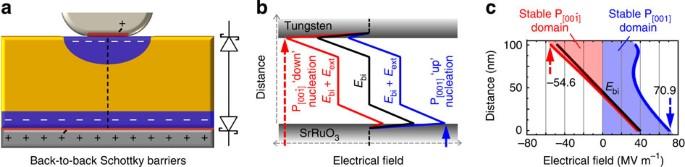Figure 3: Electrical properties of the metal-ferroelectric-metal structure. (a) A schematic of the distribution of space charge corresponding to the formation of two depletion regions and (b) the corresponding built-in electric field (black line labelledEbi) formed by the Shottky junctions. Additional external fieldsEextadd toEbi. The largest positive field and negative field occur on opposite interfaces preferentially nucleating up and down domains, respectively. (c) The electric-field accounting for the tip-effect on the external electric field. The curves correspond to 0 V (black), +0.4 V (red) and −4.8 V (blue). In reality, E ext from the W tip decreases rapidly with distance from the contact point so the curves in Figure 3b should appear more as illustrated in Figure 3c and Supplementary Figure S3 . In the case that the brief room temperature W/PZT contact does not reach chemical equilibrium and fully form the predicted Schottky junction, the tip-enhanced electric field still explains the single site P [00[macr1]] domain nucleation at the surface probe contact point. Figure 3: Electrical properties of the metal-ferroelectric-metal structure. ( a ) A schematic of the distribution of space charge corresponding to the formation of two depletion regions and ( b ) the corresponding built-in electric field (black line labelled E bi ) formed by the Shottky junctions. Additional external fields E ext add to E bi . The largest positive field and negative field occur on opposite interfaces preferentially nucleating up and down domains, respectively. ( c ) The electric-field accounting for the tip-effect on the external electric field. The curves correspond to 0 V (black), +0.4 V (red) and −4.8 V (blue). Full size image The asymmetry in switching speed between the positive and negative branches can also be ascribed to the built-in fields at the interfaces. Maksymovych et al . [13] have correlated asymmetric piezoresponse hysteresis loops in ferroelectric BiFeO 3 films to random-field defects, including built-in junction potentials. Notably, they show that random-field defect induced reduction in nucleation bias also corresponds to a decrease in the switching speed. This can be intuitively explained in the context of the slow switching observed here during the negative branch whose total electric field resembles the red curve in Figure 3c . At the time of nucleation, the electric field exceeds the coercive field only at the interface, but rapidly decreases with depth, crossing zero mid-film below which the domain is not thermodynamically favoured. 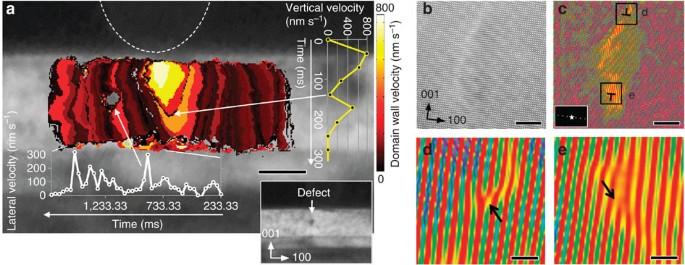Figure 4: Domain wall velocities and defect pinning. (a) A contour map of the domain outline at each time step with the colour corresponding to the domain wall velocity. Line profiles for the initial vertical velocity and lateral velocity versus time of the left domain wall are overlaid. In both cases, a pinning event is highlighted by a white arrow. Scale bar, 50 nm. (b) A high-resolution high-angle annular dark-field image of a defect (labelled in the inset ina) corresponding to the pinned region of the lateral domain wall. (c) The same image filtered in Fourier space (inset) by including only the (h00) lattice plane frequencies. Scale bars, 5 nm (bandc). The labelled ‹100›adislocation cores are magnified in panelsdande(scale bars, 1 nm). The domain wall velocity is dependent on the applied electric field, hence its velocity can be expected to decrease quickly after nucleation, which is born out in a domain wall velocity contour plot in Figure 4a , taken from the previously discussed negative switching event. The forward propagation of the domain is momentarily halted between the third and fourth time steps, labelled by a white arrow from the minimum in the corresponding vertical velocity versus time curve inset at right, possibly a result of collision with the zero-field crossover. The positive branch, in contrast, has an electric field profile shown by the blue curve in Figure 3c . At the time of nucleation the domain is thermodynamically stable through the entire film thickness, hence, switching is rapid. Figure 4: Domain wall velocities and defect pinning. ( a ) A contour map of the domain outline at each time step with the colour corresponding to the domain wall velocity. Line profiles for the initial vertical velocity and lateral velocity versus time of the left domain wall are overlaid. In both cases, a pinning event is highlighted by a white arrow. Scale bar, 50 nm. ( b ) A high-resolution high-angle annular dark-field image of a defect (labelled in the inset in a ) corresponding to the pinned region of the lateral domain wall. ( c ) The same image filtered in Fourier space (inset) by including only the (h00) lattice plane frequencies. Scale bars, 5 nm ( b and c ). The labelled ‹100› a dislocation cores are magnified in panels d and e (scale bars, 1 nm). Full size image The role of single defects can be explored in this cyclic switching data by making use of the presence of an interior segment of a threading dislocation off center to the tip contact (inset in Fig. 4a ). The lateral expansion of both the P [00[macr1]] and P [001] domains in the previously discussed switching branches interact with this dislocation during their respective switching cycles. A high-resolution HAADF image of the threading dislocation in Figure 4b shows the distorted region, which is bounded by two misfit dislocations, each with Burgers vectors ‹100›. Figure 4c shows the Fourier-filtered image using 200 reflections with the dislocation cores labelled. They are shown magnified in Figure 4d (top) and Figure 4e (bottom). The influence of this defect on the domain wall can be observed by comparing the lateral domain wall velocities of the left and right domain walls during the negative switching branch ( Figs 2c and 4a ). When the left domain wall nears the dislocation there is a sudden spike in the domain wall velocity to 300 nm s −1 as it jumps toward the defect position, manifested as a bright red band in the velocity map in Figure 4a and as a sharp peak in the inset lateral velocity versus time curve. There is no corresponding spike mirrored on the right edge of the expanding domain, ruling out a change in bias or surface contact. For 233 ms after the spike, the domain wall velocity lies in a trough, never exceeding 50 nm s −1 , which is manifested as a dark band left of the dislocation. This initial attraction towards and resistance past the dislocation loop indicates a weak pinning of the 180° domain-wall to the defect. The regions of compressive and tensile stress are mirrored by the pair of dislocations, and cancel when averaged along the domain wall plane ruling out significant net piezoelectric or flexoelectric effects. The vertical 180° domain-wall itself is neither ferroelastic nor charged, precluding strong elastic or electrostatic interactions with the dislocation. This suggests that the pinning is the result of an energy reduction by having coincident regions of disorder. Defect pinning is further demonstrated by the positive branch of the switching cycle. The left edge of the backswitched P [001] domain is consistently coincident with the dislocation ( Fig. 2b ). This pinning manifests in a clear disparity between the lateral velocities ( Fig. 2d ) and the degree of switching reversal of the left (pinned) and right domain walls. The strength of the pinning is potentially larger during this positive branch as the domain walls are heavily inclined, causing them to be positively charged due to head-to-head polarization vectors normal to the domain wall. This allows for additional electrostatic interactions with ionized dopants or polar defects that may have diffused to the dislocation core. Although 180° switching is typical of c-oriented tetragonal ferroelectric materials, stronger defect pinning through elastic interactions would be expected from ferroelastic switching paths such as 90° switching in a tensile strained film or from 71° or 109° switching in a rhombohedral ferroelectric. Despite the proximity of the dislocation to the tip, nucleation and growth kinetics appear to be dominated by the respective interfaces. Especially on the negative branch, the presence of a defect on one side of the domain does not appear to produce a significant lateral domain asymmetry. The large regional variations observed in switching kinetics are therefore likely due to interface effects, either surface defects modifying the local nucleation energy or heterogeneous screening or doping modifying the local built-in fields. Such questions will be the purview of future in situ TEM studies on the role of structural and compositional variations on ferroelectric switching. Materials synthesis and characterization A 50 nm epitaxial SRO layer was deposited as a bottom electrode on a single crystal (110)o DyScO 3 substrate by 90° off-axis sputtering at 630 °C [20] . A total pressure of 200 mTorr was maintained during deposition with a 3:2 ratio of Ar and O 2 gas. Epitaxial 100 nm PZT films were grown on top of the SRO bottom electrode by 90° off-axis sputtering at 530 °C. A mixture of Ar and O 2 gas with a 1:1 ratio was used with a total pressure of 200 mTorr. Cross-sectional TEM samples were prepared by conventional mechanical polishing followed by argon ion milling. TEM experiments were carried out using JEOL 2010F and spherical-aberration-corrected TEMs: JEOL 2100F at University of Michigan and FEI Titan 80–300 (TEAM 0.5) at Lawrence Berkeley National Laboratory. In situ TEM In situ experiments were carried out using a Nanofactory scanning tunnelling microscopy platform for TEM. Electrical bias was applied between an electrochemically etched tungsten tip, used as a movable surface electrode, and the conductive buffer layer SRO bottom electrode, which was connected to the holder ground using silver paint. The resulting capacitor structure is depicted schematically in Figure 1a . External voltages were applied using an HP 6614c for DC voltages and an HP 3324a function generator for triangle waveforms. The domain structure was imaged in realtime by using the reflection, g =202 p (the subscript p denotes pseudocubic indices), as labelled in the SAED pattern in Supplementary Figure S1b . The Supplementary Movies were recorded by a (Gatan) TV-rate camera at 29 frames per second. Domain geometries were determined in Matlab using thresholded contrast changes as follows: −30 for the positive and +20 for the negative branch out of a 1-byte pixel depth. Domain wall velocities were determined by finding the domain wall positions using a least-squares fit of first- and second-order polynomials to the domain edges determined by the Prewitt edge detection algorithm. Model and values used for the electric field calculations PZT is typically a p-type semiconductor with a band gap of ~3.4 eV, electron affinity of ~3.5 eV and work function of ~5.8 eV [29] . The work function of tungsten is about 4.5 eV [28] and SRO's is ~4.9 eV [30] . Owing to the higher work function of PZT compared with tungsten and SRO, Schottky barriers are formed at the tungsten/PZT and SRO/PZT interfaces causing the depletion of carriers at the interface and band bending (energy diagram in Supplementary Fig. S2a ). The built-in electric field produced by the ionized dopants reaches its maximum value of at the interfaces ( Supplementary Fig. S2b ). For the 100 nm film a homogeneous dopant concentration in excess of 5×10 19 cm −3 leads the film to be fully depleted of carriers, in which case it contains a homogeneous built-in space charge [30] resulting in the energy diagram and fields in Supplementary Figure S2c,d . Using the values above, the estimated built-in barriers are 1.3 and 0.9 V at the interfaces of tungsten/PZT and SRO/PZT, respectively, as shown in Supplementary Figures S2a and c . This corresponds to built-in electrical fields of 47.6 and 39.6 MV m −1 at the interfaces of tungsten/PZT and SRO/PZT, respectively, ( Supplementary Fig. S2d ). Application of an external bias to the tungsten/PZT/SRO heterostructure changes the distribution of space charge affecting the built-in electrical field. We calculated the distribution of electrical fields in PZT using Ansoft Maxwell software for finite element analysis. All calculations assume a tip diameter of ~50 nm, SRO and tungsten as perfect conductors and PZT as a perfect insulator with a resistivity of ~10 7 Ω m and relative dielectric constant of ~10 3 (ref. 31 ). Given a bias of −4.8 V, the distribution of external electrical field is shown in Supplementary Figure S3a . The distribution is inhomogeneous because of the geometrically asymmetric conductors. To estimate the electrical field at the interface in the presence of external bias, we computed the built-in potential distribution and its derivative, the electrical field, along the film normal directly beneath the tip. The estimated profile of the total electric field was determined by superposition of the applied and built-in electric fields as shown for multiple voltages given a 50-nm diameter tip ( Supplementary Fig. S3b ). This treatment is an illustrative first approximation of the actual potential distribution. The true built-in fields depend on surface states, thermal history of the electrode interfaces and the electrical history of the sample due to charge injection and the domain orientation and structure (depolarizing fields due to bound charges at the ferroelectric surfaces). The applied field is also dependent on the specific tip geometry, surface contact, sample history and the dominant conduction mechanism. How to cite this article: Gao, P. et al . Revealing the role of defects in ferroelectric switching with atomic resolution. Nat. Commun. 2:591 doi: 10.1038/ncomms1600 (2011).